Smoking exacerbates amyloid pathology in a mouse model of Alzheimer’s disease Several epidemiological studies have shown that cigarette smoking might alter the incidence of Alzheimer’s disease. However, inconsistent results have been reported regarding the risk of Alzheimer’s disease among smokers. Previous studies in experimental animal models have reported that administration of some cigarette components (for example, nicotine) alters amyloid-β aggregation, providing a possible link. However, extrapolation of these findings towards the in vivo scenario is not straightforward as smoke inhalation involves a number of other components. Here, we analysed the effect of smoking under more relevant conditions. We exposed transgenic mouse models of Alzheimer’s disease to cigarette smoke and analysed the neuropathological alterations in comparison with animals not subjected to smoke inhalation. Our results showed that smoking increases the severity of some abnormalities typical of Alzheimer’s disease, including amyloidogenesis, neuroinflammation and tau phosphorylation. Our findings suggest that cigarette smoking may increase Alzheimer’s disease onset and exacerbate its features and thus, may constitute an important environmental risk factor for Alzheimer’s disease. Alzheimer’s disease (AD) is the most common type of senile dementia in the elderly population. Histopathologically, AD is characterized by the extracellular accumulation of misfolded amyloid-β (Aβ) into senile plaques and the formation of neurofibrillary tangles, which are filamentous intracellular inclusions formed by hyperphosphorylated tau. Other AD lesions include a massive inflammatory response, characterized by activated microglia and reactive astrocytes, synaptic impairment and neuronal loss in selective areas of the brain [1] , [2] . The aetiology of sporadic AD is not well known, but several risk factors have been shown to increase the probability of developing the disease [3] . Although the main risk factor for AD is aging, various others factors have also been proposed, including gender, ApoE polymorphism, the coexistence of other disorders (such as cardiovascular diseases, brain injury, diabetes and Down syndrome) and several lifestyle conditions, including physical activity, education, diet or smoking [4] , [5] . The effects of smoking on AD remain unclear. For many years, smoking was considered to be protective for the development of AD [6] , [7] . It was proposed that acute stimulation of neuronal nicotinic receptors may have beneficial effects on people with AD [8] and that prolonged treatment may have further benefits by increasing neuronal survival [9] . Furthermore, it was reported that nicotine can decrease amyloid precursor protein (APP) secretion in animal models [10] , [11] , inhibit acquisition of β-sheet conformation by Aβ peptide [12] , diminish its aggregation [13] , reduce β-amyloidosis [14] and prevent memory impairment [15] . In fact, cotinine, the main metabolite of nicotine, is able to reduce Aβ deposition by inhibiting its oligomerization and decrease memory impairment in transgenic AD mice [16] . Moreover, some studies have found that smoking is able to reduce Aβ42 levels both in control and AD patients [17] . However, more recent epidemiological studies have demonstrated that smoking could increase the risk of AD [18] , [19] , [20] , [21] . A detailed risk assessment study concluded that ~14% of AD cases are potentially attributable to smoking, and thus a 25% reduction in smoking frequency could potentially lower AD prevalence by many hundred thousand cases worldwide [3] . Moreover, histopathological studies showed that smokers have more severe neuropathological alterations than those who have never smoked, including neurofibrillary changes and neuritic plaques [22] , [23] . To explain the discrepancy in the results, it was proposed that the deleterious effect of smoking on AD may have been masked by the fact that subjects who would have subsequently developed AD had either died or left the study due to other co-morbidities [24] , [25] . From the mechanistic viewpoint, it has been reported that nicotine exacerbates tau phosphorylation both in mouse and rat models of AD [26] , [27] . In addition, it has also been described that smoking can directly induce cognitive impairment [28] , [29] . In the present study, we investigated the effects of smoking on amyloid burden, inflammatory response, tau phosphorylation and neurodegeneration in the hippocampus and cortical area in a double-transgenic mouse model of AD. We found that smoking exacerbates Alzheimer’s-like pathology in this in vivo model of AD. Cigarette smoke in APP/PS1 increases blood cotinine levels APP/PS1 transgenic mice were exposed to both mainstream (smoke inhaled by an active smoker) and sidestream smoke (smoke from the burning end of a cigarette) in a non-ventilated exposure chamber, using a peristaltic pump that sucked the smoke from the cigarette with an airflow rate of 80 ml min −1 ( Fig. 1 ). Smoke from a commercially available cigarette was administrated 5 days per week in two different doses for 4 months. Treatment started when the animals were 3 months of age and they were sacrificed at the age of 7 months for analysis. The high-dose group received the smoke of one cigarette during 60 min, whereas low dose group received half of a cigarette during 30 min. Control transgenic animals were exposed to room air only. To measure the amount of smoke taken by the mice, we analysed the levels of cotinine in plasma during the treatment. Cotinine, the primary metabolite of nicotine, is used as a biomarker for cigarette smokers and those exposed to environmental tobacco smoke due to its longer half-life compared with that of nicotine [30] . In passive smokers, cotinine level in plasma is ~4.4 ng ml −1 , whereas for active smokers, it is >10 ng ml −1 (ref. 31 ), even after the administration of low-nicotine cigarettes [32] . Cotinine levels in plasma could reach up to 500 ng ml −1 in heavy smokers. As cotinine is completely cleared from the system after 3 days of smoke exposure, we quantified cotinine levels in plasma after 1, 2 and 3 days of treatment in low-dose and high-dose groups to check the exposure level to tobacco smoke ( Fig. 2 ). The high dose group reaches the cotinine levels of a light active smoker (>10 ng ml −1 ) 3 days after starting smoke administration, whereas the low dose group displays a cotinine concentration of <5 ng ml −1 ( Fig. 2 ). These cotinine values suggest that mice receiving low dose of cigarette smoke uptake a similar amount of smoke as passive smokers, whereas mice treated under the high dose of cigarette smoke receive a similar exposure as light active smokers. 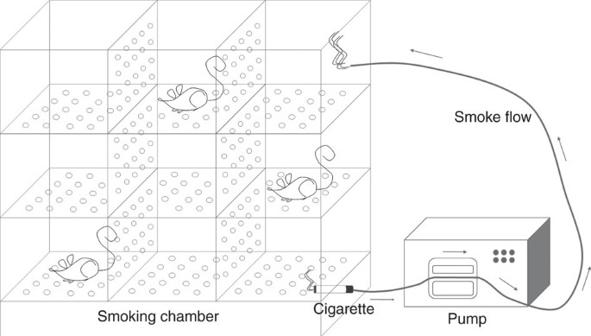Figure 1: Diagram of the smoking chamber and smoke flow. A peristaltic pump was used to suck the smoke from the cigarette and redirect it into the chamber again. Both mainstream and sidestream smoke was put into the chamber. The smoking chamber has nine compartments connected by holed panels. During the treatment, the animals were rotated for a more homogeneous cigarette-smoke exposure. No animals were placed on the compartments that directly received the smoke (either from the cigarette or from the pump). Control animals were exposed only to room air in a similar chamber. Figure 1: Diagram of the smoking chamber and smoke flow. A peristaltic pump was used to suck the smoke from the cigarette and redirect it into the chamber again. Both mainstream and sidestream smoke was put into the chamber. The smoking chamber has nine compartments connected by holed panels. During the treatment, the animals were rotated for a more homogeneous cigarette-smoke exposure. No animals were placed on the compartments that directly received the smoke (either from the cigarette or from the pump). Control animals were exposed only to room air in a similar chamber. 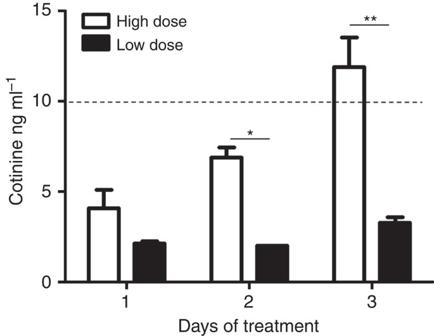Figure 2: Mice exposed to high dose of cigarette smoke contain comparable amounts of cotinine in serum as light active smokers. The level of cotinine in blood provides a direct quantification of the nicotine intake and is thus, a valuable indicator of tobacco smoke exposure31. Low-dose-treated animals showed a low cotinine blood level, which is in the range observed for passive smokers (<10 ng ml−1); whereas in high-dose-treated animals, cotinine blood levels were similar to light active smokers (>10 ng ml−1). The significance of the differences was evaluated by two-way ANOVA, followed by individual comparison using Bonferroni post test. Data are shown as mean (±s.e.m.).n=3 animals/group; *P<0.05; **P<0.01. Full size image Figure 2: Mice exposed to high dose of cigarette smoke contain comparable amounts of cotinine in serum as light active smokers. The level of cotinine in blood provides a direct quantification of the nicotine intake and is thus, a valuable indicator of tobacco smoke exposure [31] . Low-dose-treated animals showed a low cotinine blood level, which is in the range observed for passive smokers (<10 ng ml −1 ); whereas in high-dose-treated animals, cotinine blood levels were similar to light active smokers (>10 ng ml −1 ). The significance of the differences was evaluated by two-way ANOVA, followed by individual comparison using Bonferroni post test. Data are shown as mean (±s.e.m.). n =3 animals/group; * P <0.05; ** P <0.01. Full size image Cigarette smoking exacerbates amyloid load and plaque density Amyloid beta (Aβ) extracellular accumulation is one of the main neuropathological features of AD. To determine whether smoking affects Aβ deposition, we analysed Aβ burden, density and size of amyloid deposits in 7-month-old control transgenic animals and those treated with different doses of cigarette smoke. We focused on the hippocampus and cortex because these regions are the most affected by amyloid deposition in AD in both humans and transgenic animals. Histological analysis of immunostained slides with a specific antibody against Aβ (4G8, which recognizes amino acid residues 17–24 of Aβ) was performed in exposed and unexposed mice ( Fig. 3 ). APP/PS1 animals start to develop amyloid plaques around 5–6 months-old [33] , [34] . At 7 months of age, the control animals and those exposed to a low dose of cigarette smoke, display a small amount of Aβ plaques in cortical ( Fig. 3a ) and hippocampal ( Fig. 3b ) regions. Quantification of Aβ burden, expressed as percentage of stained area per total area analysed, showed a significant increase (>33%) in amyloid load in high-dose-treated animals compared with the low-dose group or the control unexposed animals in the cerebral cortex ( n =5–6 animals/group, four sections per animal; P =0.016 by one-way one-way analysis of variance (ANOVA); P <0.05 by post-hoc Tukey’s multiple comparisons test) ( Fig. 3c ). However, despite a trend, amyloid burden was not significantly increased in the hippocampal region by smoke exposure ( Fig. 3d ). The increase of amyloid load could be related with an increase in the number of plaques, the size of the amyloid deposits, or both. To address this question, we next quantified the density of amyloid plaques and expressed this measurement as the number of amyloid plaques per mm 2 . In this case, we found significant differences in plaque density in both cortex ( Fig. 3e ) and hippocampus ( Fig. 3f ) (+39.7% and +48.6%, respectively). These results indicate that smoke exposure exacerbates the pathology by increasing the amount of amyloid plaques, possibly by promoting the formation of new plaques. To further investigate this issue, we studied the size distribution of amyloid deposits, classifying them into four different size ranges: plaques <200 μm 2 , 200–500 μm 2 , 500–1,000 μm 2 and >1,000 μm 2 . In both cortex ( Fig. 3g ) and hippocampus ( Fig. 3h ), we observed a significant increase in the number of small plaques (+53.0% and +60.5% respectively) in the high-dose group compared with that in the low-dose and control groups ( n =5–6 animals/group, four sections per animal; P =0.035 by two-way ANOVA; P <0.05 and P <0.01 by post-hoc test, respectively). This result suggests that the primary effect of tobacco smoke on amyloid is to promote the formation of new Aβ deposits. 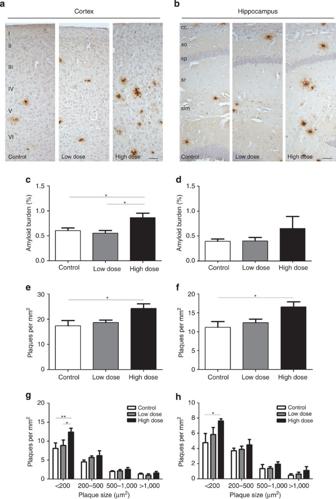Figure 3: Smoking significantly increases Aβ load and amyloid plaque density in animals exposed to high-dose cigarette smoke. Light microscopic images of 4G8-immunoreactivity counterstained with hematoxylin in cortex (a) and hippocampus (b) of control, low-dose and high-dose cigarette smoke-treated mice. Image analysis was done to estimate the amyloid burden in cortex (c) and hippocampus (d), which is expressed as the percentage of the area reactive with anti-Aβ antibody in relation to the total area analysed. The amyloid plaque density (number of plaques per area) was also calculated in both cortex (e) and hippocampus (f). The size distribution of plaques in cortex (g) and hippocampus (h) was determined to investigate whether smoke exposure has a differential effect on plaque formation or growth. I–VI: cortical layers; cc: corpus callosum; so: stratum oriens; sp: stratum pyramidale; sr: stratum radiatum; slm: stratum lacunosum moleculare. Data (mean±s.e.m.) was analysed by one-way (c–f) or two-way (g–h) ANOVA followed by Tukey’s multiple comparisons post test. Significance (*P<0.05; **P<0.01) was indicated in the figure.n=5–6 animals/group, four sections per animal. Scale bar: 50 μm. Figure 3: Smoking significantly increases Aβ load and amyloid plaque density in animals exposed to high-dose cigarette smoke. Light microscopic images of 4G8-immunoreactivity counterstained with hematoxylin in cortex ( a ) and hippocampus ( b ) of control, low-dose and high-dose cigarette smoke-treated mice. Image analysis was done to estimate the amyloid burden in cortex ( c ) and hippocampus ( d ), which is expressed as the percentage of the area reactive with anti-Aβ antibody in relation to the total area analysed. The amyloid plaque density (number of plaques per area) was also calculated in both cortex ( e ) and hippocampus ( f ). The size distribution of plaques in cortex ( g ) and hippocampus ( h ) was determined to investigate whether smoke exposure has a differential effect on plaque formation or growth. I–VI: cortical layers; cc: corpus callosum; so: stratum oriens; sp: stratum pyramidale; sr: stratum radiatum; slm: stratum lacunosum moleculare. Data (mean±s.e.m.) was analysed by one-way ( c – f ) or two-way ( g – h ) ANOVA followed by Tukey’s multiple comparisons post test. Significance (* P <0.05; ** P <0.01) was indicated in the figure. n =5–6 animals/group, four sections per animal. Scale bar: 50 μm. Full size image To evaluate the influence of smoking in the formation of fibrillar amyloid deposits, Thioflavin-S (ThS) staining was done in sections corresponding to the cortical area ( Fig. 4a ), hippocampus ( Fig. 4b ) and subiculum ( Fig. 4c ). Quantification of ThS-positive fibrillar amyloid shows that high-dose-treated animals display a larger amount of these structures in both cortex (+58.1%) and hippocampus (+103.0%) ( Fig. 4d and e ) compared with low-dose-treated animals and controls ( n =5–6 animals/group, four sections per animal; P =0.021 and P =0.041 respectively by one-way ANOVA; P <0.05 by post-hoc test). However, the ThS-positive amyloid burden in the subicular area was not significantly different among groups after smoke exposure ( Fig. 4f ). These results indicate that smoking can also enhance the maturation of amyloid plaques. Alternatively, it is also possible that smoking can stimulate the earlier deposition of plaques, giving them more time to mature. Therefore, exposure to high-dose cigarette smoke induces an increase in the number, burden and maturation of amyloid plaques in hippocampus and cortex. No significant effect on any of these parameters was observed when the animals were subjected to low doses of cigarette smoke, comparable to those received by passive smokers. 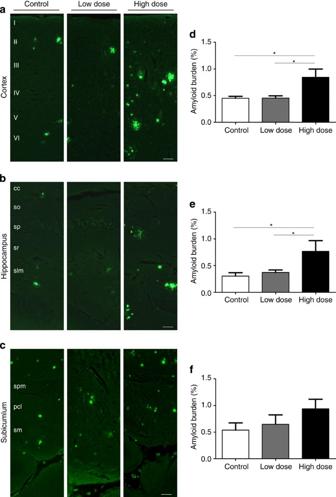Figure 4: Fibrillar Aβ load is significantly increased in high-dose smoke treated-animals. Epifluorescent microscopic images of ThS staining shown in cortex (a), hippocampus (b), and subiculum (c) of control, low-dose and high-dose cigarette smoke-treated mice. The burden of ThS-positive amyloid plaques was increased in high-dose-treated mice in both cortical areas (d) and hippocampus (e) compared with control and low-dose age-matched mice. However, no significant changes were observed in the subicular area (f). I–VI: cortical layers; cc: corpus callosum; so: stratum oriens; sp: stratum pyramidale; sr: stratum radiatum; slm: stratum lacunosum molecular; spm: stratum polymorphic; pcl: pyramidal cell layer; sm: stratum moleculare. Data (mean±s.e.m.) was analysed by one-way ANOVA followed by Tukey’s multiple comparison test (n=5–6 animals/group, four sections per animal). Scale bar: 50 μm. *P<0.05. Figure 4: Fibrillar Aβ load is significantly increased in high-dose smoke treated-animals. Epifluorescent microscopic images of ThS staining shown in cortex ( a ), hippocampus ( b ), and subiculum ( c ) of control, low-dose and high-dose cigarette smoke-treated mice. The burden of ThS-positive amyloid plaques was increased in high-dose-treated mice in both cortical areas ( d ) and hippocampus ( e ) compared with control and low-dose age-matched mice. However, no significant changes were observed in the subicular area ( f ). I–VI: cortical layers; cc: corpus callosum; so: stratum oriens; sp: stratum pyramidale; sr: stratum radiatum; slm: stratum lacunosum molecular; spm: stratum polymorphic; pcl: pyramidal cell layer; sm: stratum moleculare. Data (mean±s.e.m.) was analysed by one-way ANOVA followed by Tukey’s multiple comparison test ( n =5–6 animals/group, four sections per animal). Scale bar: 50 μm. * P <0.05. Full size image Enhancement of neuroinflammation by cigarette smoking Another important hallmark of AD pathology is a chronic inflammatory response in the brain associated with amyloid deposition. This neuroinflammatory process manifests as an increase of reactive astrocytes and activated microglia [35] . To determine the effect of cigarette smoke in AD-associated microglial activation, we immunostained microglial cells using Iba1 antibody ( Fig. 5a-d ) and quantified the labelled area in relation to the total area analysed. Iba1 is a protein specifically expressed in microglial cells with macrophage activity and is upregulated during their activation [36] . As noticed in the representative pictures, both cortex ( Fig. 5a ) and hippocampus ( Fig. 5b ) display lower Iba1-inmmunoreactivity in control animals and low-dose-treated animals compared with the high dose group. Activated microglial cells in the control group (arrow in Fig. 5c ) are scattered and less abundant than in the high-dose group, where enlargement of the cell body and swelling of microglial processes is highly prominent (arrows in Fig. 5d ). Most of the microglial cells are arranged in clusters, probably surrounding the plaques. The densitometric analysis of light microscopic images showed an enhanced microglial activation in high-dose-treated animals compared with low-dose and control groups in both cortex (+50.0%) and hippocampus (+85.7%) ( n =5–6 animals/group, four sections per animal; P =0.032 and P =0.028 respectively by one-way ANOVA; P <0.05 by post-hoc test) ( Fig. 5e and f ). To evaluate whether microglial activation was due to amyloid deposition, we analysed the correlation between microglial and amyloid staining in all the studied groups. The Pearson correlation coefficient value was 0.72 ( P <0.0001), indicating a significant positive correlation between amyloid burden and microglial activation. 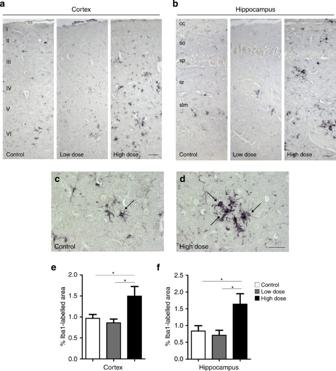Figure 5: Microglial activation is significantly increased in high-dose smoke-treated animals. Light microscopic images of Iba1-immunoreactivity (specific for microglial cells) shown in cortex (a) and hippocampus (b) of control, low-dose and high-dose cigarette smoke-treated mice. Higher magnification images of Iba1-staining show the increased number of hypertrophied activated microglial cells (arrows ind) that appear in the cortex of the high-dose-treated animals compared with the control group (c). Activated microglial cells were statistically increased in high-dose-treated mice in both cortical (e) and hippocampal (f) areas compared with low-dose and untreated age-matched mice. I–VI: cortical layers; cc: corpus callosum; so: stratum oriens; sp: stratum pyramidale; sr: stratum radiatum; slm: stratum lacunosum moleculare. Data (mean±s.e.m.) was analysed by one-way ANOVA followed by Tukey’s multiple comparisons test.n=5–6 animals/group, four sections per animal. Scale bar: 50 μm (a–b), 25 μm (c–d). *P<0.05. Figure 5: Microglial activation is significantly increased in high-dose smoke-treated animals. Light microscopic images of Iba1-immunoreactivity (specific for microglial cells) shown in cortex ( a ) and hippocampus ( b ) of control, low-dose and high-dose cigarette smoke-treated mice. Higher magnification images of Iba1-staining show the increased number of hypertrophied activated microglial cells (arrows in d ) that appear in the cortex of the high-dose-treated animals compared with the control group ( c ). Activated microglial cells were statistically increased in high-dose-treated mice in both cortical ( e ) and hippocampal ( f ) areas compared with low-dose and untreated age-matched mice. I–VI: cortical layers; cc: corpus callosum; so: stratum oriens; sp: stratum pyramidale; sr: stratum radiatum; slm: stratum lacunosum moleculare. Data (mean±s.e.m.) was analysed by one-way ANOVA followed by Tukey’s multiple comparisons test. n =5–6 animals/group, four sections per animal. Scale bar: 50 μm ( a – b ), 25 μm ( c – d ). * P <0.05. Full size image We also wanted to determine the effect of cigarette smoke exposure in astrogliosis. Astroglial cells were immunostained using GFAP antibody ( Fig. 6a–d ), which recognizes an intermediate filament protein (glial fibrillary acidic protein) expressed mainly in astrocytes. GFAP immunostaining was highly increased in the high-dose-exposed group compared with that in the control and low dose groups, as shown in representative pictures of the cortical ( Fig. 6a ) and hippocampal ( Fig. 6b ) areas. Higher magnification of reactive astrocytes in the cortex is shown for the control ( Fig. 6c ) and high-dose group ( Fig. 6d ). Numerous reactive astrocytes with cell body hypertrophy and thickened processes were seen in the high-dose-treated group (arrows in Fig. 6d ) compared with that in the control group. Results of densitometric analysis showed a significant increase in the area occupied by reactive astrocytes in cortex (+105.0%) and hippocampus (+71.1%) of high-dose-treated animals compared with low-dose and control animals ( Fig. 6e and f ) ( n =5–6 animals/group, four sections per animal; P =0.014 and P =0.009 respectively by one-way ANOVA; P <0.05 by post-hoc tests). The correlation between astroglial immunostaining and amyloid deposition was determined by linear regression. The Pearson correlation coefficient value was 0.67 ( P <0.0001), indicating a significant positive correlation between the two variables including all studied groups. These results indicate that animals exposed to high doses of tobacco smoke exhibit a higher inflammatory response in hippocampus and cortex, and that this neuroinflammatory process is likely the result of higher amyloid deposition induced by smoking. 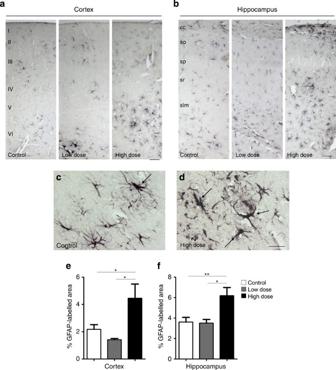Figure 6: Reactive astrogliosis is augmented in high-dose smoke-treated animals. Light microscopic images of GFAP-immunoreactivity (specific for astroglial cells) shown in cortex (a) and hippocampus (b) of control, low-dose and high-dose cigarette smoke-treated mice. High magnification images of GFAP-stained reactive astroglial cells (arrows) in the cortical area of control (c) and high-dose groups (d). Immunostained astrocytes were increased in high-dose-treated mice in both cortical area (e) and hippocampus (f) compared with control and low-dose age-matched mice. I–VI: cortical layers; cc: corpus callosum; so: stratum oriens; sp: stratum pyramidale; sr: stratum radiatum; slm: stratum lacunosum moleculare. Data (mean±s.e.m.) was analysed by one-way ANOVA followed by Tukey’s multiple comparisons test.n=5–6 animals/group, four sections per animal. Scale bar: 50 μm (a–b), 25 μm (c–d). **P<0.01; *P<0.05. Figure 6: Reactive astrogliosis is augmented in high-dose smoke-treated animals. Light microscopic images of GFAP-immunoreactivity (specific for astroglial cells) shown in cortex ( a ) and hippocampus ( b ) of control, low-dose and high-dose cigarette smoke-treated mice. High magnification images of GFAP-stained reactive astroglial cells (arrows) in the cortical area of control ( c ) and high-dose groups ( d ). Immunostained astrocytes were increased in high-dose-treated mice in both cortical area ( e ) and hippocampus ( f ) compared with control and low-dose age-matched mice. I–VI: cortical layers; cc: corpus callosum; so: stratum oriens; sp: stratum pyramidale; sr: stratum radiatum; slm: stratum lacunosum moleculare. Data (mean±s.e.m.) was analysed by one-way ANOVA followed by Tukey’s multiple comparisons test. n =5–6 animals/group, four sections per animal. Scale bar: 50 μm ( a – b ), 25 μm ( c – d ). ** P <0.01; * P <0.05. Full size image Tau phosphorylation is increased in smoke-treated animals It is well known that the presence of amyloid deposits produces an increase in cellular oxidative stress, which leads to a dysregulation in the activity of serine/threonine kinases, among others [37] . These kinases are involved in tau phosphorylation, inducing its hyperphosphorylation, which presumably leads to tangle formation [38] . To determine whether smoke exposure modulates tau phosphorylation, we analysed tau hyperphosphorylation by using a phospho-specific anti-tau antibody, AT8, which recognizes phosphorylation in Ser-202 and Thr-205 (ref. 39 ) [39] , costained with ThS to label amyloid plaques ( Fig. 7 ). Representative pictures of cortical plaques are shown. Whereas in non-treated animals, no significant AT8-positive staining was found ( Fig. 7a ); small punctuated AT8-positive staining, similar to dystrophic neurites, appear in the low- and high-dose groups both in cortex and hippocampal areas, mainly surrounding amyloid plaques ( Fig. 7b and c ). Although the low dose group demonstrated very little AT8-immunoreactivity (arrow in Fig. 7b2 ), AT8-positive staining was evident in high-dose-treated animals, exhibiting tau hyperphosphorylation surrounding most of the amyloid plaques (arrows in Fig. 7c2 ). At this point, we cannot determine if this increase in tau phosphorylation is due to a direct effect of smoking treatment or due to the higher amount of amyloid plaques. It is important to highlight that the observed tau alterations are far from the neuritic tau pathology seen in AD brain. However, it is widely known in the field that bona-fide tau pathology is not seen in mice, unless animals express human mutant tau. 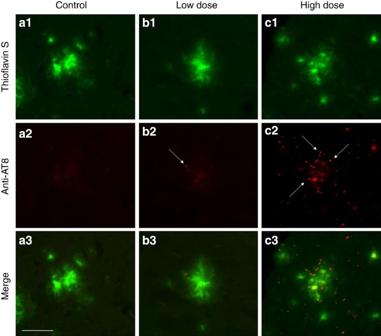Figure 7: Abnormally phosphorylated tau is enhanced in smoke-treated animals. Representative epifluorescent microscopic images of ThS staining (green) and anti-AT8 phosphorylated tau antibody (red) seen in control (a1–a3), low-dose (b1–b3) and high-dose (c1–c3) cigarette smoke-treated mice in the motor cortex. High-dose smoking induces tau hyperphosphorylation (arrows inc2) compared with control and low-dose age-matched mice, in which little or no AT8-positive staining was found. Abnormally phosphorylated tau accumulates mainly around amyloid plaques (c3). Scale bar: 25 μm. Figure 7: Abnormally phosphorylated tau is enhanced in smoke-treated animals. Representative epifluorescent microscopic images of ThS staining (green) and anti-AT8 phosphorylated tau antibody (red) seen in control ( a1 – a3 ), low-dose ( b1 – b3 ) and high-dose ( c1 – c3 ) cigarette smoke-treated mice in the motor cortex. High-dose smoking induces tau hyperphosphorylation (arrows in c 2) compared with control and low-dose age-matched mice, in which little or no AT8-positive staining was found. Abnormally phosphorylated tau accumulates mainly around amyloid plaques ( c 3). Scale bar: 25 μm. Full size image Neurodegeneration is not affected by cigarette smoke Neuronal death is a common feature during aging and in neurodegenerative diseases, such as AD. Several transgenic models of AD recapitulate some of the neuropathological alterations observed in AD patients, but they scarcely show any evidence of neuronal death [40] . To evaluate whether neurodegeneration is also enhanced by exposure to cigarette smoke, we analysed neuronal loss by quantifying the number of neurons in cortex, hippocampus and subiculum after staining with NeuN antibody, which recognizes a neuron-specific protein in mature neurons ( Fig. 8a–c ). No significant differences were found in neuronal density among the three groups in the cortical area ( Fig. 8d ), CA1–CA3 hippocampal areas ( Fig. 8e ) or subiculum ( Fig. 8f ). The lack of differences in neurodegeneration among the groups was also confirmed by Fluoro-Jade C staining, which labels specifically degenerating neurons (data not shown). Nevertheless, it is still possible that some particular subsets of neurons could be specifically vulnerable to cigarette-smoke exposure. 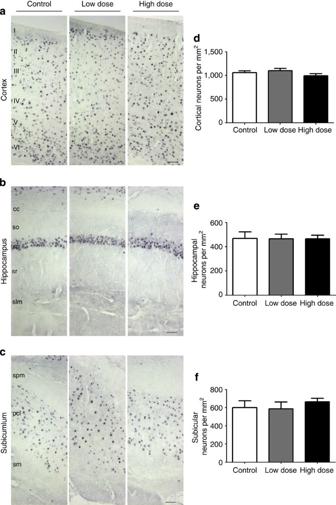Figure 8: Neurodegeneration is not modified by smoking exposure. Neuronal density (number of neurons per mm2) was estimated by quantifying the number of neurons after NeuN staining (a-c). Neuronal density is similar in control and smoke-exposed animals (P>0.5) in cortical region (d), CA1–CA3 hippocampal areas (e) and subiculum (f) positing that cigarette smoke does not increase the rate of neuronal death. I–VI: cortical layers; so: stratum oriens; sp: stratum pyramidale; sr: stratum radiatum; spm: stratum polymorphic; pcl: pyramidal cell layer; sm: stratum moleculare. Data (mean±s.e.m.) was analysed by one-way ANOVA test.n=5–6 animals/group. Scale bar: 50 μm. Figure 8: Neurodegeneration is not modified by smoking exposure. Neuronal density (number of neurons per mm 2 ) was estimated by quantifying the number of neurons after NeuN staining ( a-c ). Neuronal density is similar in control and smoke-exposed animals ( P >0.5) in cortical region ( d ), CA1–CA3 hippocampal areas ( e ) and subiculum ( f ) positing that cigarette smoke does not increase the rate of neuronal death. I–VI: cortical layers; so: stratum oriens; sp: stratum pyramidale; sr: stratum radiatum; spm: stratum polymorphic; pcl: pyramidal cell layer; sm: stratum moleculare. Data (mean±s.e.m.) was analysed by one-way ANOVA test. n =5–6 animals/group. Scale bar: 50 μm. Full size image Sporadic, late-onset AD is the most common form of the disease, which is likely associated with a complex set of environmental and genetic risk factors. Based on epidemiological studies and in vitro and in vivo experiments with nicotine administration, it was initially proposed that smoking might be protective against AD [6] , [7] , [12] , [13] , [14] . However, more recent and complete demographic studies have shown that smoking represents one of the largest risk factors for AD [3] , [19] , [20] , [21] , [22] . To study the effect of cigarette smoking on the onset of brain alterations typical of AD, we exposed mice, genetically engineered to develop some of the neuropathological features of AD, to complete tobacco smoke, under similar conditions in which smokers are exposed to this material. Double transgenic APP/PS1 mice expressing two of the human genes associated with AD were exposed to different doses of cigarette smoke, 5 days per week, during 4 consecutive months. The pathological features of AD were measured and compared with the untreated control counterparts. Our results suggest that smoking increases amyloid deposition in a dose-dependent manner, by promoting the formation of new plaques and contributing to the maturation of amyloid deposits. Smoking also exacerbates gliosis, inducing microglial activation and reactive astrogliosis in the mice exposed to high doses of smoke. Neuroinflammatory response was exacerbated after smoke exposure and correlated with the increase of amyloid lesions. Exposure to smoke also induced alterations in tau phosphorylation around the amyloid plaques, which are considered a precursor of tangle formation. However, we could not find a decrease in neuronal density in smoke-exposed animals. Our findings provide direct evidence that cigarette smoking exacerbates some of the typical neuropathological alterations associated with AD in vivo . The mechanisms by which smoking increases the risk of AD abnormalities remain unclear. There are several possible pathways by which smoking may have this deleterious effect, including direct induction of protein misfolding and aggregation due to some of the smoking components, increase of oxidative stress, impairments of the proteostasis machinery, cerebrovascular damage, brain inflammation and so on. Further studies are needed to elucidate which of these different mechanisms operate and whether the same effect is also observed in humans. Our results suggest that cigarette smoking may contribute to the accumulation of cerebral protein aggregates and, thus, may constitute an important environmental risk factor for AD and other protein misfolding diseases. Transgenic mice APPswe/PS1dE9 (B6C3-Tg (APPswe, PSEN1dE9) 85Dbo/J, The Jackson Laboratory) double transgenic mice express a chimeric mouse/human amyloid precursor protein containing the Swedish mutation (Mo/HuAPP695swe) and a mutant human presenilin 1 (PS1dE9) gene. The generation and initial characterization of these mice has been reported previously [34] . APP/PS1 animals develop amyloid deposits by 5–6 months old mostly located in the hippocampus, cortex and subiculum and display behavioural impairment by 13 months of age. Animals were housed in groups of up to five in individually ventilated cages under standard conditions (22 °C, 12 h light–dark cycle) receiving food and water ad libitum . All animal experiments were carried out in accordance with the NIH regulations. Cigarette smoke exposure Two groups of male and female APP/PS1 transgenic animals ( n =5–6/group) were each subjected to two separate smoking exposure conditions during 4 months. Transgenic mice were subjected to both mainstream and sidestream smoke obtained from a commercial brand using a specially designed non-ventilated chamber containing a peristaltic pump that sucked the smoke from the cigarette with an airflow rate of 80 ml min −1 ( Fig. 1 ). In the high-dose treatment, transgenic mice were exposed daily (5 days per week) for 60 min to the smoke generated from one cigarette. A second group of mice received a low dose of smoke defined as 30 min in the smoking chamber containing the smoke of half a cigarette. Control animals were exposed to room air in an identical chamber. Treatment started at the age of 3 months, and animals were sacrificed at 7 months of age, when amyloid plaques started to appear in this model. Cotinine determination in blood Exposure to tobacco smoke can be detected by measuring nicotine metabolites (for example, cotinine) in blood, as cotinine has a longer half-life than nicotine. Cotinine plasma levels were measured by using a competitive mouse/rat cotinine ELISA kit (Calbiotech). Blood samples were obtained via tail venipuncture 1 h before, and 1, 2 and 3 days after smoke exposure (immediately after exposure). To obtain plasma samples, blood was collected in EDTA-coated tubes and centrifuged at 2,000 × g for 20 min. Plasma was separated and stored at −80 °C until use. Proteins from the plasma fraction were loaded directly onto ELISA plates and treated according to the manufacturer’s recommendations. Samples were loaded in duplicate, and absorbance was read at 450 nm on an ELISA plate reader (EL800, BioTek). Immunohistochemistry The mice were killed by CO 2 inhalation and perfused transcardially with PBS. Brains were removed, post-fixed into fixative solution (10% neutral buffered formalin) and embedded in paraffin. Serial sections (1 out of 10 sections) from all animal groups ( n =5–6 per group; four sections per stain per animal) were processed in parallel for immunostaining using the same solutions to minimize variability in staining conditions. Deparaffinized 10-μm-thick sections were used for immunohistochemical staining. After blocking the endogenous peroxidase activity with 3% H 2 O 2 –10% methanol in PBS, pH 7.4 for 20 min, the sections were incubated overnight at room temperature in one of the primary antibodies: mouse anti-4G8 (1:1,000 Covance); rabbit anti-Iba1 (1:1,000 Wako); rabbit anti-GFAP (1:1,000 Abcam); mouse anti-ptau (1:100 AT8, Pierce); or rabbit anti-NeuN (1:1,000 Millipore). Primary antibody was detected by incubating 1 h with the corresponding HRP-linked secondary antibody: sheep anti-mouse or donkey anti-rabbit (1:1,000 GE Healthcare). Peroxidase reaction was visualized using DAB Kit (Vector) following the manufacturer’s instructions. For counterstaining, the sections were incubated in Harris hematoxylin for 1 min (Fisher). Finally, the sections were dehydrated in graded ethanol, cleared in xylene and coverslipped with DPX mounting medium and examined under a bright field microscope (DMI6000B, Leica). Fluorescent staining For ThS (Sigma) staining, the sections were incubated in ThS solution (0.025% in 50% ethanol) for 5 min after deparaffinization, rinsed, coverslipped with mounting medium for fluorescence (Vector) and immediately visualized using a fluorescence microscope. For double AT8/Thioflavin-S fluorescent labelling, the sections were first incubated with the primary antibody followed by Alexa594-conjugated secondary antibody. Then, the sections were washed and processed for Thioflavin-S staining and coverslipped with mounting medium for fluorescence to avoid photobleaching. Fluoro-Jade C (FJC) (Millipore) staining was done to detect degenerating neurons. The sections were deparaffinized and immersed in basic alcohol (1% sodium hydroxide in 80% ethanol) for 5 min. After rinsing in 70% ethanol and distilled water, the slides were incubated in 0.06% potassium permanganate solution for 10 min, washed and incubated for 10 min in 0.0001% FJC solution and dissolved in 0.1% acetic acid. Finally, the sections were dehydrated and covered with DPX mounting medium and examined under an epifluorescent microscope (DMI6000B, Leica). Plaque size morphometric analysis and burden quantification Four sagittal serial sections stained with 4G8 antibody from each group were analysed using ImageJ 1.45s software for plaque size morphometry. Burden quantification was done through the lateromedial extent of the cortical and hippocampal areas in the sagittal plane (between 0.70 and 1.60 mm lateral to the midline), being the first section of each animal randomly collected. Quantification was assessed in every tenth section (with a distance of 100 μm among them), and four 10 μm sections were measured in each animal ( n =5–6/group). Brain boundaries were defined according a standard mouse stereotaxic brain atlas, and 10 × objective was used for individual plaque measurement. Number of plaques per mm 2 falling into four surface categories (ranging from <200 μm 2 to >2,000 μm 2 ) was calculated. Photomicrographs were taken by using a DFC310 FX Leica digital camera (Leica), imported into ImageJ 1.45s software (NIH) and converted to black and white images. The threshold intensity was manually set and kept constant, and the number of pixels was determined for 4G8-, ThS-, Iba1- and GFAP stained sections to quantify amyloid load, fibrillar burden, microglial activation and reactive astrogliosis in hippocampal (CA1, CA2, CA3 and dentate gyrus), subiculum and cortical areas (including motor, somatosensory, visual, frontal, parietal and retrosplenial cortex). Amyloid plaque density was performed manually using the same software by calculating the area and the number of plaques per total analysed area. Each analysis was done by a single examiner blinded to sample identities. Neuronal density analysis The number of NeuN-immunopositive cells was counted using a bright field microscope (DMI6000B, Leica) 20 × objective. Photomicrographs were taken by using a DFC310 FX Leica digital camera and imported into ImageJ 1.45 s software (NIH). Quantification was done semi-automatically. The images were converted to black and white images, threshold intensity was set, and the number of particles was analysed by circularity. Cell counting was done through the lateromedial extent of the cortical and hippocampal areas in the sagittal plane (between 0.70 and 1.60 mm lateral to the midline), including CA1, CA2 and CA3 areas of the hippocampus, subiculum and cortical areas (motor, somatosensory, visual, frontal, parietal and retrosplenial cortex). As previously described, neurons were quantified in every tenth section, and four 10 μm sections were measured in each animal ( n =5–6/group). Brain boundaries were defined according a standard mouse stereotaxic brain atlas. The numerical density is expressed as neurons per mm 2 . An investigator who was blind to the experiment performed neuronal profile counting. Statistical analysis Graphs are expressed as means±s.e.m. After confirming normal distribution with skewness and kurtosis statistic test, ANOVA followed by a post-hoc Tukey’s multiple comparisons test were used to analyse differences among groups. For the size distribution analysis of plaques, we applied two-way ANOVA followed by Bonferroni test. Statistical analyses were performed using GraphPad Prism 5.0 software (GraphPad Software). For linear correlation, Pearson correlation coefficient was used. Statistical differences for all tests were considered significant at the P <0.05 level. How to cite this article: Moreno-Gonzalez, I. et al . Smoking exacerbates amyloid pathology in a mouse model of Alzheimer’s disease. Nat. Commun. 4:1495 doi: 10.1038/ncomms2494 (2013).